NOG1increases grain production in rice During rice domestication and improvement, increasing grain yield to meet human needs was the primary objective. Rice grain yield is a quantitative trait determined by multiple genes, but the molecular basis for increased grain yield is still unclear. Here, we show that NUMBER OF GRAINS 1 ( NOG1 ), which encodes an enoyl-CoA hydratase/isomerase, increases the grain yield of rice by enhancing grain number per panicle without a negative effect on the number of panicles per plant or grain weight. NOG1 can significantly increase the grain yield of commercial high-yield varieties: introduction of NOG1 increases the grain yield by 25.8% in the NOG1 -deficient rice cultivar Zhonghua 17, and overexpression of NOG1 can further increase the grain yield by 19.5% in the NOG1 -containing variety Teqing. Interestingly, NOG1 plays a prominent role in increasing grain number, but does not change heading date or seed-setting rate. Our findings suggest that NOG1 could be used to increase rice production. Rice ( Oryza sativa L.), one of the earliest domesticated crops, feeds over one-third of the population in the world as a staple food [1] . During the evolutionary course of cultivated rice from wild rice ( Oryza rufipogon Griff. ), marked morphological changes have occurred. In recent years, several key genes, which control the critical transitions of morphological traits such as seed shattering, prostrate growth habit, grain color, the spreading panicle, and awn development, have been isolated in rice [2] , [3] , [4] , [5] , [6] , [7] , [8] , [9] , [10] , [11] , [12] , [13] , [14] , [15] . The transition from less grain number per panicle to a greater number per panicle (Fig. 1 a, b) is one of the most important events in rice domestication. After the domestication, further selection would occur for pursuing high-yield production, which could meet the needs for food as the global population increases. Grain yield of rice is a complicated trait and is directly determined by three main components, including the number of panicles per plant, the number of grains per panicle, and grain weight. In recent years, several genes controlling yield-related traits have been characterized [16] , [17] , [18] , [19] , [20] , [21] , [22] , [23] , [24] , [25] , [26] , [27] , [28] , [29] , [30] . However, the molecular mechanisms increasing the grain yield during rice improvement are still largely unknown. Fig. 1 Comparison of a phenotype. a , b The transition of grain number from wild rice ( Oryza rufipogon ) to cultivated rice ( Oryza sativa ). A panicle is shown in the lower corner, respectively. c The main panicle of SIL176 and Guichao 2. Scale bars, 5 cm. d , e Comparison of the number of grains per main panicle and grain yield per plant between SIL176 and Guichao 2. Data are means, with error bars showing the standard error of mean (SEM), n = 30 (two-tailed Student’s t test; ** P < 0.01) Full size image Here, we report the identification of a gene, NUMBER OF GRAINS 1 ( NOG1 ), which regulates grain number and the yield of rice. We find that NOG1 encodes an enoyl-CoA hydratase/isomerase (ECH), a key enzyme in fatty acid β-oxidation pathway, and upregulation of NOG1 transcript levels significantly enhances grain number and yield without negative effects in the number of panicles, grain weight, seed-setting rate, and heading date. The identification of NOG1 will not only enhance our understanding for the molecular basis of regulation of grain yield, but will also provide a favorable gene for breeding high-yield rice. Cloning of NOG1 We identified an introgression line SIL176 with less grain number and low grain yield, which carried six introgressed segments from Dongxiang common wild rice (DXCWR, O. rufipogon Griff.) in a high-yielding indica variety Guichao 2 background [31] (Supplementary Fig. 1 ). Compared with Guichao 2, grain number per main panicle and grain yield per plant of SIL176 decreased by 39.6% and 44.3%, respectively (Fig. 1c–e ). Phenotype observations found that primary branch number, grain number of primary branches, the secondary branch number, and grain number of secondary branches of SIL176 were significantly less than those of Guichao 2 (Supplementary Fig. 2a–d ). However, no significant differences were observed in the number of panicles per plant, 1000-grain weight, seed-setting rate, and heading date between SIL176 and Guichao 2 (Supplementary Fig. 2e–h ). The F 1 plants from the cross between SIL176 and Guichao 2 displayed similar phenotypes of grain number per main panicle and grain yield per plant to Guichao 2 (Supplementary Fig. 2i, j ). A genetic linkage analysis of 243 F 2 individuals derived from the cross between SIL176 and Guichao 2 showed that there is a major QTL, NOG1 , which locates between SSR markers RM1183 and RM297 on chromosome 1, and explains 13% of phenotypic variance of grain number per main panicle and 12% of phenotypic variance of grain yield per plant. 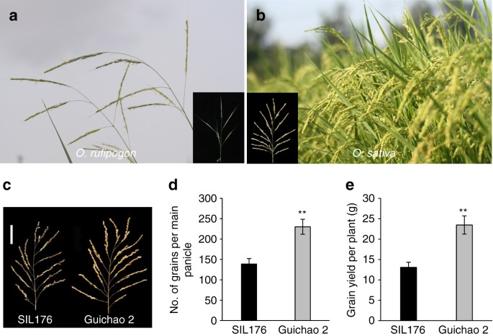Fig. 1 Comparison of a phenotype.a,bThe transition of grain number from wild rice (Oryza rufipogon) to cultivated rice (Oryza sativa). A panicle is shown in the lower corner, respectively.cThe main panicle of SIL176 and Guichao 2. Scale bars, 5 cm.d,eComparison of the number of grains per main panicle and grain yield per plant between SIL176 and Guichao 2. Data are means, with error bars showing the standard error of mean (SEM),n= 30 (two-tailed Student’sttest; **P< 0.01) The allele from Guichao 2 at the locus could increase the grain number per main panicle and grain yield per plant (Supplementary Table 1 ). To score the phenotype precisely and conveniently, we selected the number of grains per main panicle as the targeted trait for fine-mapping NOG1 . Progeny test of 6230 F 2 individuals derived from the cross between Guichao 2 and SIL176 revealed that NOG1 was delimited to a 4.3-kb region between the single-nucleotide polymorphism (SNP) marker 860CX5 and 870CX2. Annotation according to the MSU Rice Genome Annotation Project Database ( http://rice.plantbiology.msu.edu/ ) showed that the 4.3-kb mapping region harbors the promoter ( cis -regulatory region) and the first three exons of LOC_Os01g54860, and the last exon of LOC_Os01g54870 (Fig. 2a ). Sequencing the 4.3-kb mapping region revealed that there was one 12-bp insertion–deletion (InDel) and 15 SNPs between Guichao 2 and SIL176 in the promoter region of LOC_Os01g54860 (Supplementary Fig. 3a Fig. 2 Mapping and cloning of NOG1 . a The NOG1 locus was detected on chromosome 1. Positional cloning narrowed the NOG1 locus to a 4.3-kb region between 860CX5 and 870CX2. The numbers above the bars indicated the number of recombinants. LOC_Os01g54860 was the candidate gene. b The main panicle of SIL176 (control), complemented transgenic plants (SIL176-CTP), and Guichao 2. Scale bars, 5 cm. c Comparison of the relative expression levels of NOG1 among SIL176, SIL176-CTP, and Guichao 2 ( n = 4). d , e Comparison of grain number per main panicle and grain yield per plant among SIL176, SIL176-CTP, and Guichao 2 ( n = 30). f The main panicle of Guichao 2 (control), RNAi transgenic plants (Guichao 2-RNAi), and SIL176. Scale bars, 5 cm. g Comparison of the relative expression levels of NOG1 among Guichao 2, Guichao 2-RNAi, and SIL176 ( n = 4). h , i Comparison of grain number per main panicle and grain yield per plant among Guichao 2, Guichao 2-RNAi, and SIL176 ( n = 30). Data are means, with error bars showing SEM (two-tailed Student’s t test; ** P < 0.01) Full size image To verify the function of LOC_Os01g54860, we generated a complementary construct (pCPL), which contained a 6903-bp fragment, including the entire gene region and 2504-bp promoter region of LOC_Os01g54860 from Guichao 2, and introduced the pCPL construct into SIL176 using Agrobacterium -mediated transformation. Compared with the SIL176 (control), relative expression levels of LOC_Os01g54860 were elevated, and grain number per main panicle and grain yield per plant were increased in the complemented transgenic plants (SIL176-CTP) (Fig. 2b–e ), but there were no changes in the number of panicles per plant, 1000-grain weight, seed-setting rate, and heading date (Supplementary Fig. 4 a–d). To further validate the function of LOC_Os01g54860, we transformed an RNA interference construct (pRNAi) into Guichao 2. We found that the LOC_Os01g54860 transcript levels reduced, and grain number per main panicle and grain yield per plant decreased in the RNAi transgenic plants (Guichao 2-RNAi) compared with control plants (Fig. 2f–i ). We also found that there were no significant differences in the number of panicles per plant, 1000-grain weight, seed-setting rate, and heading date between transgenic plants and control (Supplementary Fig. 4e–h ). Taken together, these results demonstrated that LOC_Os01g54860 is NOG1 that is essential for regulating the grain number per panicle and grain yield per plant in rice. Transcriptional characterization of NOG1 Sequence analysis of 5′- and 3′-rapid amplification of complimentary DNA (cDNA) ends (RACE) and cDNA products indicated that the NOG1 cDNA in Guichao 2 is 1479-bp long, with an open reading frame of 1167-bp, a 159-bp 5′-untranslated region, and a 153-bp 3′-untranslated region, and it encodes a 388-amino-acid protein (Supplementary Fig. 3b ). We constructed a vector harboring NOG1-GFP (green fluorescence protein) fusion gene driven by a CaMV35S promoter, and then introduced a plasmid into onion epidermal cells and rice protoplast cells. The fluorescent signal showed that the NOG1 protein was localized in the nucleus and cytoplasm (Fig. 3a–d ). Fig. 3 Transcriptional characterization of NOG1 . a – d The subcellular localization of NOG1 protein. a , b The p35S :: GFP and p35S :: NOG1-GFP fusion gene were transiently expressed in onion inner epidermal cells. Scale bars, 100 μm. c , d Subcellular localization of the p35S :: GFP and p35S :: NOG1-GFP fusion gene in rice protoplast cells. Scale bars, 5 μm. The NOG1-GFP protein was localized in both the nucleus and the cytosol. e The expression pattern of NOG1 in SIL176 and Guichao 2. Expression analysis of NOG1 in root, tiller base, culm, eustipes, pulvinus, leaf, and young panicles. Data are means, with bars showing SEM, n = 3. (two-tailed Student’s t test; ** P < 0.01). f – h Expression patterns analysis of NOG1 revealed by messenger RNA (mRNA) in situ hybridization during panicle development in Guichao 2. f Sense probes as negative controls. Scale bars, 100 μm; g RNA in situ hybridization of NOG1 during panicle development. Scale bars, 100 μm; h Enlarged from g marked by a red square. Scale bars, 20 μm. i – k Expression patterns analysis of NOG1 revealed by mRNA in situ hybridization during panicle development in SIL176. i Sense probes as negative controls. Scale bars, 100 μm; j RNA in situ hybridization of NOG1 during panicle development. Scale bars, 100 μm; k Enlarged from j marked by a red square. Scale bars, 20 μm Full size image We investigated the tissue specificity of NOG1 expression using real-time quantitative PCR (RT-qPCR). The results showed that NOG1 expression was detected in various rice organs, including root, tiller base, culm, eustipes, pulvinus, leaf, and young panicles, and NOG1 relative expression levels in the leaf and young panicles of Guichao 2 were significantly higher than that of SIL176 (Fig. 3e ). At the same time, the expression levels of F 1 plants in young panicles were similar with Guichao 2, consistent with a phenotype (Supplementary Fig. 2k ). RNA in situ hybridization signals of NOG1 in young panicles indicated that NOG1 is expressed in the primordia of branches, and hybridization signals in Guichao 2 were stronger than that in SIL176 (Fig. 3f–k ). The high levels of NOG1 expression in developing panicles are consistent with its role in controlling the grain number in rice. A 12-bp insertion enhances NOG1 expression and grain number Sequence analysis showed that there was one 12-bp InDel (ATGGCAACTTTG) and 15 SNP variations in the promoter region of NOG1 between SIL176 and Guichao 2 (Fig. 4a ). Interestingly, there are two closely connected copies of the 12-bp, which locates the 2214-bp upstream of the translation start site in Guichao 2, but there is only one copy of the 12-bp in SIL176. Further analysis of the promoter of NOG1 using a database of Plant Cis-acting Regulatory DNA Elements (PLACE, www.dna.affrc.go.jp/PLACE/signalup.html ), showed that there are two transcription factor-binding sites (TFBS) within the 12-bp InDel, one is DOFCOREZM (−) AAAG (DOF TFBS) and another is TBOXATGAPB (+) ACTTTG. Fig. 4 Association test and expression profile of NOG1 variation. a Sequences comparison of a promoter region between SIL176 and Guichao 2. b Association testing with grain number per main panicle of 16 variants in the 4.3-kb fine-mapping region. Black dots represent 16 variations. c Triangle matrix of pairwise linkage disequilibrium. d Effect of the 12-bp insertion and 15 SNPs in NOG1 promoter by transient expression assays. Above, constructs of pGreenII 0800- LUC vector. Left, constructs with site-directed NOG1 promoter. SIL176 and Guichao 2 define the constructs with the ~2500-bp promoter fragments from SIL176 and Guichao 2, respectively. The SIL176 promoter contained one copy of the 12-bp and the 15 SNPs-type 1 (ACTTCTAATCCAGAG). The Guichao 2 promoter contained two copies of the 12-bp and the 15 SNPs-type 2 (TGCCTAGCCTTGTTA). A1, A2, and A3 define constructs with site-directed mutations at the 12-bp InDel (positions −2214) and 15 SNPs (positions from −2166 to −405) in the SIL176 promoter fragment, respectively. A4 and A5 define constructs with site-directed mutations at TBOXATGAPB and DOFCOREZM TFBS on the 12-bp InDel in the SIL176 promoter fragment, respectively. Right, expression levels of firefly luciferase relative to Renilla luciferase ( n = 10). e Comparison of NOG1 gene expression levels between varieties containing one copy of 12-bp and varieties containing two copies of 12-bp ( n = 20). Data are means, with error bars showing SEM (two-tailed Student’s t test; ** P < 0.01) Full size image To determine the relationships between the mutations in the NOG1 promoter region and the grain number, we sequenced the 4.3-kb fine-mapping region of 158 cultivars, including 84 indica and 74 japonica varieties. An association test between grain number per main panicle and sequence variations in the promoter region showed that the strongest signal was present at the 12-bp InDel and 7 SNPs (Fisher’s exact test, P < 0.01) (Fig. 4b, c ). To verify whether the 12-bp InDel and 15 SNPs in the NOG1 promoter region affected the NOG1 gene expression, we generated constructs by installing mutant promoter fragments into the binary vector pGreenII 0800- LUC , and introduced the constructs into rice protoplasts for transient expression assays. Compared with the transient relative activity of the SIL176 promoter, the relative activities of mutant promoter fragment with 15 SNP variations but without 12-bp InDel (A3 construct) did not change. It suggested that 15 SNPs have no impact on the expression of NOG1 gene. Furthermore, deletion of the 12-bp (A1 construct) and mutation of DOF TFBS in 12-bp (A5 construct) significantly reduced the transcriptional activity of the SIL176 promoter. Adding one copy of 12-bp (A2 construct) enhanced the transcriptional activity of the SIL176 promoter, as well as the Guichao 2 promoter (Fig. 4d ). To further verify whether the 12-bp InDel was responsible for the regulation of NOG1 gene expression, 20 cultivars containing two copies of 12-bp and 20 cultivars containing one copy of 12-bp were selected to investigate their NOG1 gene expression. The results showed that the expression levels of NOG1 gene in these varieties containing two copies of 12-bp were obviously higher than that in varieties containing one copy of 12-bp (Fig. 4e ). The results suggest that the 12-bp insertion with DOF TFBS in the NOG1 promoter region might be responsible for the NOG1 expression levels among rice accessions. To ascertain whether expression levels of NOG1 affect the grain number, we generated the overexpression construct harboring nog1 cDNA from SIL176, driven by the maize ubiquitin promoter. The construct was introduced into an elite japonica rice variety Zhonghua 17 that harbors the nog1 cDNA identical to SIL176. Compared with Zhonghua 17 as a control, NOG1 expression was significantly enhanced, and grain number per panicle and grain yield per plant were significantly increased in the overexpression transgenic plants (Supplementary Fig. 5 ). The results indicated that upregulation of the NOG1 expression levels could increase the grain number per panicle and grain yield per plant in rice. Taken together, the 12-bp insertion in the NOG1 promoter region upregulates the NOG1 expression, resulting in the increase of grain number and grain yield in rice. NOG1 expression affects the ECH levels A protein-BLAST (BLASTp) at NCBI online and gene identification by MSU-RGAP revealed that NOG1 encodes an ECH that catalyzes a reversible syn-hydration of trans -2,3-enoyl-CoA to the corresponding L-3-hydroxyacyl-CoA [32] . Compared with the nog1 cDNA of SIL176, NOG1 cDNA of Guichao 2 has a 3-bp deletion on the 14th exon, resulting in an amino-acid deletion after being translated (Supplementary Fig. 3c, d ). To verify whether the NOG1/nog1 protein has ECH activity, the NOG1/nog1 protein was encoded by NOG1 / nog1 -coding sequence from Guichao 2/SIL176, driven by the AOX1 promoter, which was eukaryotic expressed in yeast Pichia pastoris . We assayed the enzyme activity of eukaryotic expression products and found that the equivalent amount of NOG1 and nog1 protein generated a similar ECH enzyme activity (Fig. 5a ). These results indicated that the NOG1 protein has ECH activity, and two proteins of NOG1 and nog1 have equal enzymatic activity; thus, the 3-bp InDel in the NOG1 -coding sequence did not affect the NOG1 protein function, which was consistent with the results that the 3-bp deletion was out of the 4.3-kb fine-mapping region. Fig. 5 Functional analysis of NOG1 . a ECH enzymatic activity assays of NOG1/nog1 and 6×His fusion protein by eukaryotic expression in Pichia yeast. The empty pPICZ-C vector plasmid was transfected as control (pPICZ), and pPICZ-GC and pPICZ-S176 were transfected by NOG1 and nog1 , respectively ( n = 10). b Enzymatic activity assays of ECH in young panicles among Guichao 2, SIL176, and transgenic plants ( n = 10). c Comparison of the total fatty acid content in young panicles among Guichao 2, SIL176, and transgenic plants ( n = 3). d – f Comparison of JA, OPDA, and JA-Ile levels in young panicles among Guichao 2, SIL176, and transgenic plants ( n = 10). g Main panicle of Guichao 2 and JA-treated Guichao 2. Scale bars, 5 cm. h , i Comparison of JA contents and the number of grains per main panicle between Guichao 2 and JA-treated Guichao 2 ( n = 10). j Comparison of NOG1 expression levels between Guichao 2 and JA-treated Guichao 2 ( n = 3). Data are means, with error bars showing SEM (two-tailed Student’s t test; ** P < 0.01; * P < 0.05; NS, P > 0.05) Full size image Further investigation of the ECH enzyme activity in young panicles showed that ECH enzyme levels both in Guichao 2 and the complemented transgenic plants (SIL176-CTP) were higher than that in SIL176, while ECH enzyme levels in the RNAi transgenic plants (Guichao 2-RNAi) were lower than that in the control plants (Guichao 2) (Fig. 5b ). These results suggested that the NOG1 expression affected the ECH enzyme levels, and upregulation of the NOG1 expression increased the ECH enzyme levels in plants. NOG1 expression regulates fatty acid β-oxidation A previous study revealed that ECH is a key enzyme in the second step of fatty acid β-oxidation pathway, and leads to component accumulation of the long-chain fatty acids [32] . In order to determine whether a change of ECH enzyme levels affected fatty acid β-oxidation system, we measured fatty acids content and their composition in young panicles, using gas-liquid chromatography analysis, and found that the total fatty acids content and linolenic acid (C18:3) in Guichao 2, and the complemented transgenic plants were lower than those in the SIL176 and the RNAi transgenic plants, respectively (Fig. 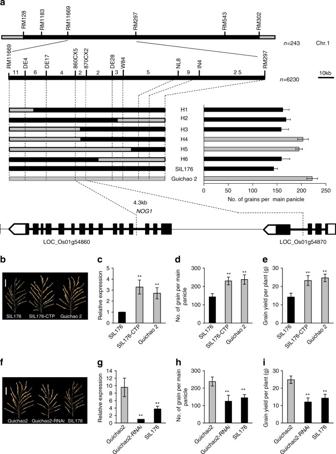Fig. 2 Mapping and cloning ofNOG1.aTheNOG1locus was detected on chromosome 1. Positional cloning narrowed theNOG1locus to a 4.3-kb region between 860CX5 and 870CX2. The numbers above the bars indicated the number of recombinants. LOC_Os01g54860 was the candidate gene.bThe main panicle of SIL176 (control), complemented transgenic plants (SIL176-CTP), and Guichao 2. Scale bars, 5 cm.cComparison of the relative expression levels ofNOG1among SIL176, SIL176-CTP, and Guichao 2 (n= 4).d,eComparison of grain number per main panicle and grain yield per plant among SIL176, SIL176-CTP, and Guichao 2 (n= 30).fThe main panicle of Guichao 2 (control), RNAi transgenic plants (Guichao 2-RNAi), and SIL176. Scale bars, 5 cm.gComparison of the relative expression levels ofNOG1among Guichao 2, Guichao 2-RNAi, and SIL176 (n= 4).h,iComparison of grain number per main panicle and grain yield per plant among Guichao 2, Guichao 2-RNAi, and SIL176 (n= 30). Data are means, with error bars showing SEM (two-tailed Student’sttest; **P< 0.01) 5c ; Supplementary Table 2 ). NOG1 decreases plant hormone jasmonic acid levels The β-oxidation pathway participates in not only the catabolism of fatty acids, but also in the metabolism of hormones and amino acids [33] . We measured the endogenous jasmonic acid (JA), 3-indoleacetic acid (IAA), and salicylic acid (SA) levels in young panicles by high-performance liquidchromatography–mass spectrometry (HPLC-MS/MS) method and found that Guichao 2 and the complemented transgenic plants showed lower endogenous JA levels, compared with SIL176 and the RNAi transgenic plants (Fig. 5d ), but there was no difference in IAA and SA levels among Guichao 2, SIL176, and transgenic plants (Supplementary Fig. 6 ). Previous studies revealed that C18:3 is the synthetic precursor of JA, and peroxisomal β-oxidation is required to convert 12-oxo-phytodienoicacid (OPDA) into JA in the last few steps of JA synthesis [34] , [35] . We examined the contents of jasmonates including OPDA and JA-isoleucine (JA-Ile) in young panicles, and compared with SIL176 and the RNAi transgenic plants, Guichao 2 and the complemented transgenic plants showed lower OPDA and JA-Ile levels, consistent with JA levels (Fig. 5e, f ). Furthermore, compared with SIL176, the expression levels of OsDAD1 , OsLOX , OsAOS2 , OsAOC , and OsOPR7 associated with JA biosynthesis pathway were downregulated in Guichao 2 (Supplementary Fig. 7a–e ). JA is one of the most important signal molecules regulating the development of plants, and higher JA levels might inhibit the development of rice spikelet and decrease grain number [36] , [37] . To further confirm whether the JA affects the grain number, we treated Guichao 2 with MeJA at the panicles development stage. After an excess of 100 mM MeJA treatment, the JA contents were increased in Guichao 2. In addition, the grain number per panicle of JA-treated Guichao 2 was decreased. Further examination showed that the NOG1 gene expression in Guichao 2 was downregulated by JA treatment (Fig. 5g–j ). These results demonstrated that the JA treatment downregulated NOG1 gene expression and decreased the grain number in rice. Origin of the NOG1 gene In order to explore the origin and distribution of the 12-bp insertion in rice, we sequenced an ~2.5-kb genomic fragment of NOG1 promoter in 158 varieties of cultivated rice and 75 accessions of wild rice. The results showed that 75 accessions of wild rice all harbor one copy of the 12-bp functional site identical to SIL176. The single copy of the 12-bp fixed in wild rice might be adaptive in the wild. However, among 158 varieties of cultivated rice, 61 varieties (48 indica and 13 japonica varieties) harbor two copies of the 12-bp functional sites identical to Guichao 2, and 97 varieties (36 indica and 61 japonica varieties) harbor one copy of 12-bp (Supplementary Tables 3 , 4 ), indicating that the mutation of the 12-bp insertion in NOG1 of cultivated rice might occur after the transition from wild rice to cultivated rice. We also found that the proportion harboring 12-bp insertion in indica varieties (57.1%) was much higher than that in japonica varieties (17.6%), suggesting that the 12-bp variation in NOG1 promoter region might have originated in the indica cultivars and was later introduced into japonica cultivars. NOG1 enhances the grain yield of rice As 61.4% of cultivars did not harbor the beneficial 12-bp insertion, we selected the commercial high-yielding japonica cultivar Zhonghua 17, which contains one copy of 12-bp, and is widely used in production. Compared with Zhonghua 17 as a control, the NOG1 -complemented transgenic plants exhibited an obvious increase in the NOG1 expression levels, grain number per panicle, and grain yield per plant, while there was no significant difference in other traits, including the number of panicles per plant, 1000-grain weight, seed-setting rate, and heading date between transgenic plants and control. Field estimation of grain yield showed that the NOG1 -complemented transgenic plants increased the grain yield by 25.8% compared with the control (Fig. 6a–e ; Supplementary Fig. 8a–d ). Fig. 6 NOG1 increases grain production in cultivars. a Grains from one plant of Zhonghua 17 (ZH17) and complemented transgenic plants (ZH-CTP). Scale bars, 5 cm. b Comparison of NOG1 expression levels between ZH17 and ZH-CTP ( n = 4). c , d Comparison of the number of grains per panicle and grain yield per plant between ZH17 and ZH-CTP ( n = 30). e Comparison of grain yield in the field between ZH17 and ZH-CTP ( n = 5). f Grains from one plant of Teqing (TQ) and NOG1 overexpression transgenic plants (TQ-OE). Scale bars, 5 cm. g Comparison of NOG1 expression levels between TQ and TQ-OE ( n = 4). h , i Comparison of the number of grains per panicle and grain yield per plant between TQ and TQ-OE ( n = 30). j Comparison of grain yield in the field between TQ and TQ-OE ( n = 5). Data are means, with error bars showing SEM (two-tailed Student’s t test; ** P < 0.01; * P < 0.05) Full size image To further explore the application potential of NOG1 in rice breeding, we introduced an overexpression construct harboring NOG1 -coding sequence into an elite commercial indica cultivar Teqing that harbors two copies of 12-bp. Compared with Teqing as a control, the expression levels of NOG1 in the transgenic plants were significantly elevated. Consistent with the high expression of NOG1 , grain number per panicle and grain yield per plant were significantly increased in the overexpression transgenic plants, while changes in other traits were not observed. Field estimation of grain yield showed that the NOG1 overexpression transgenic plants increased the grain yield by 19.5% compared with the control (Fig. 6f–j ; Supplementary Fig. 8e–h ). These results indicated that upregulating NOG1 expression can further increase the grain yield in NOG1 -containing high-yield varieties. Here, we show that the NOG1 gene can increase the grain number and yield. NOG1 encodes an enoyl-CoA hydratase/isomerase, and a 12-bp insertion in the promoter region upregulates the NOG1 gene expression, elevates the levels of the enoyl-CoA hydratase, decreases the total fatty acids and linolenic acid contents, downregulates endogenous JA levels, and enhances the grain number to increase grain yield in rice. 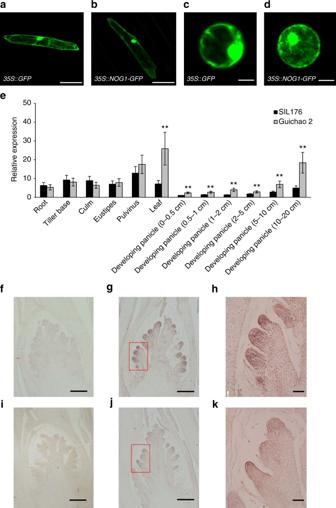Fig. 3 Transcriptional characterization ofNOG1.a–dThe subcellular localization of NOG1 protein.a,bThep35S::GFPandp35S::NOG1-GFPfusion gene were transiently expressed in onion inner epidermal cells. Scale bars, 100 μm.c,dSubcellular localization of thep35S::GFPandp35S::NOG1-GFPfusion gene in rice protoplast cells. Scale bars, 5 μm. The NOG1-GFP protein was localized in both the nucleus and the cytosol.eThe expression pattern ofNOG1in SIL176 and Guichao 2. Expression analysis ofNOG1in root, tiller base, culm, eustipes, pulvinus, leaf, and young panicles. Data are means, with bars showing SEM,n= 3. (two-tailed Student’sttest; **P< 0.01).f–hExpression patterns analysis ofNOG1revealed by messenger RNA (mRNA) in situ hybridization during panicle development in Guichao 2.fSense probes as negative controls. Scale bars, 100 μm;gRNA in situ hybridization ofNOG1during panicle development. Scale bars, 100 μm;hEnlarged fromgmarked by a red square. Scale bars, 20 μm.i–kExpression patterns analysis ofNOG1revealed by mRNA in situ hybridization during panicle development in SIL176.iSense probes as negative controls. Scale bars, 100 μm;jRNA in situ hybridization ofNOG1during panicle development. Scale bars, 100 μm;kEnlarged fromjmarked by a red square. Scale bars, 20 μm A field test showed that introduction of NOG1 increases the grain yield by 25.8% in the NOG1 -deficient rice cultivar Zhonghua 17, and overexpression of NOG1 can further increase the grain yield by 19.5% in the NOG1 -containing variety Teqing. NOG1 can significantly increase the grain yield of commercial high-yield varieties, which serves as a favorable gene to increase rice production. During the process of rice domestication from wild rice to cultivated rice, not only the morphological characters changed greatly, but also the grain yield of cultivated rice was improved significantly compared with its progenitors. Previous studies revealed that the transitions of morphological traits, such as seed shattering, prostrate growth habit, grain color, the spreading panicle, and awn development, are controlled by one or a few of the genes, respectively [2] , [3] , [4] , [5] , [6] , [7] , [8] , [9] , [10] , [11] , [12] , [13] , [14] , [15] , and the differences of grain yield between wild and cultivated rice are controlled by a lot of QTLs [38] , [39] . However, only a few genes that controlled yield improvement have been identified. 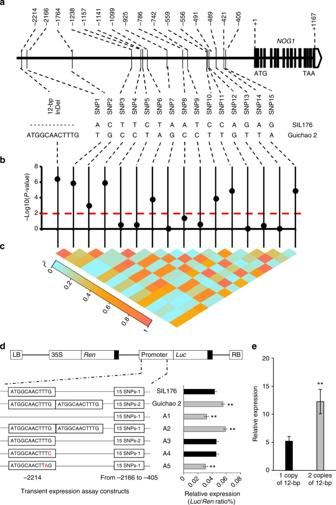Fig. 4 Association test and expression profile ofNOG1variation.aSequences comparison of a promoter region between SIL176 and Guichao 2.bAssociation testing with grain number per main panicle of 16 variants in the 4.3-kb fine-mapping region. Black dots represent 16 variations.cTriangle matrix of pairwise linkage disequilibrium.dEffect of the 12-bp insertion and 15 SNPs inNOG1promoter by transient expression assays. Above, constructs of pGreenII 0800-LUCvector. Left, constructs with site-directedNOG1promoter. SIL176 and Guichao 2 define the constructs with the ~2500-bp promoter fragments from SIL176 and Guichao 2, respectively. The SIL176 promoter contained one copy of the 12-bp and the 15 SNPs-type 1 (ACTTCTAATCCAGAG). The Guichao 2 promoter contained two copies of the 12-bp and the 15 SNPs-type 2 (TGCCTAGCCTTGTTA). A1, A2, and A3 define constructs with site-directed mutations at the 12-bp InDel (positions −2214) and 15 SNPs (positions from −2166 to −405) in the SIL176 promoter fragment, respectively. A4 and A5 define constructs with site-directed mutations at TBOXATGAPB and DOFCOREZM TFBS on the 12-bp InDel in the SIL176 promoter fragment, respectively. Right, expression levels of firefly luciferase relative to Renilla luciferase (n= 10).eComparison ofNOG1gene expression levels between varieties containing one copy of 12-bp and varieties containing two copies of 12-bp (n= 20). Data are means, with error bars showing SEM (two-tailed Student’sttest; **P< 0.01) In this study, we identify a key gene NOG1 that increases the grain number of cultivated rice. Sequence analysis showed that some cultivars, both of indica and japonica varieties still harbor one copy of 12-bp, similar to wild rice. The introduction of NOG1 increases the grain yield by ~25% in the NOG1 -deficient variety, suggesting that NOG1 is a key gene regulating the improvements of yield. Identification of NOG1 provides not only molecular evidences for yield improvements, but also a favorable gene to increase rice production. A change in the protein product caused by sequence variation on the gene-coding region is the most important molecular basis of allelic variation. However, changes of gene expression levels caused by the sequence variation on transcriptional regulatory region were also an important genetic basis of trait variation. Typical examples are OsLG1 in rice, tb1 in maize, and fw2.2 in tomato [10] , [40] , [41] , and the phenotypic changes are due to the sequence variation of their promoter regions. In this study, we find that a 12-bp repetition containing DOF TFBS in the NOG1 promoter region results in an increase of the NOG1 expression levels, leading to increasing the grain number. DOF protein is one kind of plant-specific transcription factor that plays an important role in a variety of physiological processes, including carbon metabolism, and recognizes the AAAG motif as a core-element sequence. Previous studies revealed that two concatenate-repeated AAAG motifs showed about a two-fold higher affinity for DNA than a probe containing one motif [42] . Overall, we speculate that the repetition of TFBS increases gene expression, resulting in increasing the grain number and enhancing grain yield. We can increase the grain yield by upregulating the NOG1 gene expression levels in rice breeding. The number of panicles per plant, the number of grains per panicle, and grain weight are the three important elements, and are also the important goals of breeding improvement. During the improvement of rice, changes in the target traits by genetic modification often lead to problematic agronomic traits associations because of pleiotropic gene effects. For example, IPA1 increases the grain number and grain weight but reduces panicle number [17] ; Ghd7 increases the grain number per panicle but delays heading date [20] ; and GW2 increases the grain size and the number of panicles per plant but delays heading date and reduces the grain number per panicle [24] . It is essential to rice breeding that we identify novel genes improving yield traits without any trade-offs for other agronomic or yield-related traits. The NOG1 gene identified in this study increases the grain number without adverse effects on the number of panicles, grain weight, seed-setting rate, and heading date. Homology analysis showed that the orthologs of NOG1 exist in various plants such as Sorghum bicolor , Zea mays , Setaria italica , Triticum aestivum , and so on (Supplementary Fig. 9 ). NOG1 homologous genes may play a similar function in different crops; thus, it could be explored for general grain crop improvement. We believe that NOG1 is a favorable gene for grain yield improvement, and the utilization of NOG1 is very helpful for breeding high-yield varieties of grain crops. Plant materials The introgression line, SIL176, was selected from ILs (BC 4 F 4 ), Dongxiang common wild rice was used as a donor, and Guichao 2 was used as a recipient. Other materials used in this study are listed in Supplementary Tables 3 , 4 , including 84 indica ( O. sativa L. ssp. indica ) varieties, 74 japonica ( O. sativa L. ssp. japonica ) varieties, and 75 accessions of wild rice. 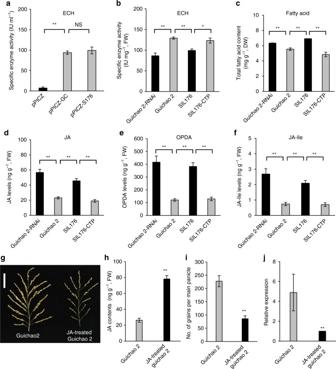Fig. 5 Functional analysis ofNOG1.aECH enzymatic activity assays of NOG1/nog1 and 6×His fusion protein by eukaryotic expression inPichiayeast. The empty pPICZ-C vector plasmid was transfected as control (pPICZ), and pPICZ-GC and pPICZ-S176 were transfected byNOG1andnog1, respectively (n= 10).bEnzymatic activity assays of ECH in young panicles among Guichao 2, SIL176, and transgenic plants (n= 10).cComparison of the total fatty acid content in young panicles among Guichao 2, SIL176, and transgenic plants (n= 3).d–fComparison of JA, OPDA, and JA-Ile levels in young panicles among Guichao 2, SIL176, and transgenic plants (n= 10).gMain panicle of Guichao 2 and JA-treated Guichao 2. Scale bars, 5 cm.h,iComparison of JA contents and the number of grains per main panicle between Guichao 2 and JA-treated Guichao 2 (n= 10).jComparison ofNOG1expression levels between Guichao 2 and JA-treated Guichao 2 (n= 3). Data are means, with error bars showing SEM (two-tailed Student’sttest; **P< 0.01; *P< 0.05; NS,P> 0.05) 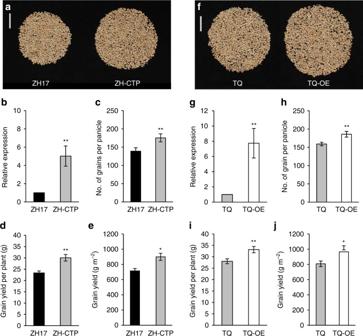Fig. 6 NOG1increases grain production in cultivars.aGrains from one plant of Zhonghua 17 (ZH17) and complemented transgenic plants (ZH-CTP). Scale bars, 5 cm.bComparison ofNOG1expression levels between ZH17 and ZH-CTP (n= 4).c,dComparison of the number of grains per panicle and grain yield per plant between ZH17 and ZH-CTP (n= 30).eComparison of grain yield in the field between ZH17 and ZH-CTP (n= 5).fGrains from one plant of Teqing (TQ) andNOG1overexpression transgenic plants (TQ-OE). Scale bars, 5 cm.gComparison ofNOG1expression levels between TQ and TQ-OE (n= 4).h,iComparison of the number of grains per panicle and grain yield per plant between TQ and TQ-OE (n= 30).jComparison of grain yield in the field between TQ and TQ-OE (n= 5). Data are means, with error bars showing SEM (two-tailed Student’sttest; **P< 0.01; *P< 0.05) Primers The primers used in this study are listed in Supplementary Table 5 . Generation of constructs and transformation of rice The 6903-bp fragment including the entire gene region and 2661-bp promoter region of NOG1 gene was amplified from Guichao 2 DNA, and was inserted into the binary vector pCAMBIA1300 to form the complementary construction pCPL. The RNAi construct pRNAi contained an inverted repeat sequence harboring the 361-bp NOG1 cDNA fragment. Two overexpression constructs pOE-GC and pOE-S176 harboring NOG1 cDNA from Guichao 2 and nog1 cDNA from SIL176, respectively, were driven by the maize ubiquitin promoter into the binary vector pCAMBIA1301. Depending on the different experimental purposes, these constructs were introduced into Agrobacterium tumefaciens strain EHA105 and subsequently transformed into SIL176, Guichao 2, Teqing, and Zhonghua 17 respectively, by Agrobacterium -mediated transformation. The phenotypes were detected in T 2 generation of transgenic plants. The testing of grain yield in the field was transplanted to 16.7 cm multiplied by 20 cm. RNA preparation and reverse transcription PCR The total RNAs were extracted from various tissues using an RNeasy Plant Mini Kit (Qiagen). First-strand cDNA was synthesized from about 2 μg of total RNAs in 20-μl volumes using Oligo (dT) 18 primer (Takara) and M-MLV reverse transcriptase (Promega). RACE and real-time quantitative PCR RACE (5’RACE and 3’RACE) were performed according to the manufacturer’s instructions of 5′-Full RACE Kit and 3′-Full RACE Core Set (Takara), respectively. RT-qPCR was done on the CFX96 Real-Time System (Bio-Rad). Diluted cDNA was amplified using the SYBR Green Master Mix (Applied Biosystems). Each set of experiments was performed on at least three plants from each line and with at least three technical replications. The rice ubiquitin gene was used as the internal control, and the measurements were obtained using the relative quantification method [43] . Subcellular localization We constructed a p35S::NOG1-GFP vector containing NOG1 -coding sequence fused with the coding sequence of GFP in a frame driven by a CaMV35S promoter, and then introduced the plasmid into onion epidermal cells and rice protoplast. The bombarded tissues were examined with a Nikon C1 confocal laser microscope. RNA in situ hybridization The freshly young panicles of Guichao 2 and SIL176 were collected and fixed in FAA solution (50 ml of ethanol, 5 ml of acetic acid, 10 ml of 37% formaldehyde, and 35 ml of DEPC-H 2 O) at 4 °C overnight, dehydration by ethanol from 50 to 100%, infiltration by xylene from 50 to 100%, and embedded in paraffin (Paraplast Plus, Fisher Scientific). The tissues were sliced into about 8–10-μm sections with a microtome (Leica RM2145), and then, the sections were mounted on RNase-free glass slides. The 192-bp 5′-region of NOG1 FL-cDNA was amplified as the template, and digoxigenin-labeled sense and antisense RNA probes were prepared using a DIG Northern Starter Kit (Roche) following the manufacturer’s instruction. RNA in situ hybridization with probes was performed on sections. Slides were observed using a microscope (Leica DMR) and photographed with a microcolor CCD camera (Apogee Instruments) [44] . Transient expression assays of promoter activity The ~2.5-kb promoter fragments upstream of the NOG1 translation start site were amplified from Guichao 2 and SIL176, respectively, and fragments with site-directed mutations at the 12-bp InDel and 15 SNPs were designed by an overlap extension of PCR. All of the fragments were inserted into pGreenII 0800- LUC . The rice protoplast was isolated from rice leaves of 7–10 days after seeding under dark conditions. Each of the NOG1 promoter– LUC gene fusion constructs was used for transient transformation into rice protoplasts. Activities of LUC to REN luciferase were measured using the Dual-Luciferase Reporter Assay System (Promega) [45] , [46] . Enzyme activity assays of ECH The coding sequence from Guichao 2 and SIL176 was inserted into eukaryotic expression vector pPICZ-C, respectively, and then two constructs and pPICZ-C empty vector plasmid as control were introduced into the yeast P. pastoris by electroporation. The ECH enzyme activity was detected by following the hydration of the double-bond band. The decrease in absorbance was measured at 263 nm, 28 °C in an assay mixture contains 0.2 mol l −1 potassium phosphate, 0.2 mg ml −1 bovine serum albumin, and 30 μmol l −1 crotonyl-CoA (Sigma) at a pH of 8.0. The extinction coefficient was using 6700 M −1 cm −1 as the calculated rate [47] . Measurements of fatty acid composition The freshly young panicles of Guichao 2, SIL176, and transgenic plants were collected and ground in liquid nitrogen. After vacuum freeze-drying process, the total fatty acid content and long-chain fatty acids compositions of samples were measured by gas–liquid chromatography analysis [48] . Measurements of endogenous hormone levels The young panicles of parental and transgenic plants were ground into powder in liquid nitrogen. Extraction and quantitative analysis of endogenous hormones from each sample (50 mg of a fresh plant tissue) was determined by high-performance liquid chromatography–mass spectrometry (HPLC–MS/MS) method [49] . MeJA treatments At 90 days after planting, before panicles initiation, Guichao 2 was subjected to 30 days until the end of panicles development, by 100 mM MeJA (95%, Sigma-Aldrich) solution. Data analysis QTL analysis was detected by the Map Manager QTX [50] . Association analysis was performed with Fisher’s exact test, as Fisher’s exact test can be powerful for qualitative traits such as grain number per panicle [51] . Multiple sequences were aligned using ClustalX [52] . A phylogenetic tree was constructed by the MEGA 5 [53] . Data availability The authors declare that the data supporting the findings of this study are available within the paper and the Supplementary Information, or are available from the corresponding author upon request. Sequence data were deposited in the GenBank under the following accession numbers: MF687920 ( NOG1 cDNA from Guichao 2) and MF687921 (DXCWR).